Telomeres are favoured targets of a persistent DNA damage response in ageing and stress-induced senescence Telomeres are specialized nucleoprotein structures, which protect chromosome ends and have been implicated in the ageing process. Telomere shortening has been shown to contribute to a persistent DNA damage response (DDR) during replicative senescence, the irreversible loss of division potential of somatic cells. Similarly, persistent DDR foci can be found in stress-induced senescence, although their nature is not understood. Here we show, using immuno-fluorescent in situ hybridization and ChIP, that up to half of the DNA damage foci in stress-induced senescence are located at telomeres irrespective of telomerase activity. Moreover, live-cell imaging experiments reveal that all persistent foci are associated with telomeres. Finally, we report an age-dependent increase in frequencies of telomere-associated foci in gut and liver of mice, occurring irrespectively of telomere length. We conclude that telomeres are important targets for stress in vitro and in vivo and this has important consequences for the ageing process. Cellular senescence is defined as the irreversible loss of division potential in somatic cells and is marked by a number of distinct phenotypic changes [1] . It is believed that senescence has an important role in vivo , protecting organisms on one hand against a build-up of cells containing DNA damage and on the other hand contributing to age-dependent tissue dysfunction [1] . Evidence is mounting that cells bearing senescent markers accumulate in several tissues with age [2] , [3] , as well as in several age-related diseases [4] , [5] . DNA damage, especially double-strand breaks (DSBs), induces a DNA damage response (DDR) [6] that leads to repair, apoptosis or permanent growth arrest (senescence). The senescent phenotype develops slowly over several days after the initial DNA damage [7] , [8] and is maintained by an ongoing DDR [7] , [9] . This response is characterized by activation of sensor kinases (ATM/ATR, DNA-PK), formation of DNA damage foci containing phosphorylated histone H2A.X (γH2A.X) and ultimately induction of checkpoint proteins, such as p53 (TP53) and the CDK inhibitor p21 (CDKN1A), which contribute to cell-cycle arrest. The described signalling pathway continues to actively contribute to the stability of the cell-cycle arrest long after induction of senescence [9] . Similar to replicative senescence, persistent DNA damage foci have also been observed as a result of stress-induced senescence induced by irradiation [7] , [8] , and while they are thought to be important in the maintenance of the phenotype, the nature of this irreparable DNA damage is still unclear. Telomeres are specialized structures at the ends of linear chromosomes, and consist of tandem TTAGGG repeats that bind proteins to form a complex named shelterin [10] . This complex sequesters the telomeric DNA and prevents it from being recognized as DNA damage [11] . Telomere-induced foci can be induced by experimental disruption of shelterin components such as TRF2 and POT1 [12] , [13] , telomere shortening during replicative senescence [9] or spontaneously in cancer cells [14] . Uncapped telomeres have been shown to become associated with DDR factors such as 53BP1, MRE11, phosphorylated forms of H2AX and ATM [12] , and activate a signalling cascade that culminates in cell-cycle arrest [9] . Telomeres are distinct from the rest of the genome in their DNA repair capacity [15] and have been shown to inhibit non-homologous end joining (NHEJ) as a mechanism to prevent end-to-end fusions [16] . NHEJ is a major pathway for the repair of DSBs, which allows the rejoining of two DNA ends and has been reported to be inhibited in vitro by shelterin components, such as TRF2 [17] . For these reasons, we speculated that telomeric repeats might be the preferential locations for unresolved DSBs, following exposure to DNA-damaging agents. The inability to repair DSBs by NHEJ at telomeric regions could be a major contributor to a persistent DDR [7] . Here, we have investigated the role of genotoxic and oxidative stress in the persistence of a DDR during cellular senescence and its potential role in mammalian ageing. We show, both by immuno-fluorescent in situ hybridization (FISH) and ChIP, that DNA damage foci in senescence induced by exogenous DNA-damaging agents are preferentially located at telomeres, irrespective of telomerase activity. Importantly, using a combination of an AcGFP-53BP1c fusion protein and telomere PNA probes in live cells, we show that all persistent foci (surviving for longer than 3 h) are associated with telomeres. Moreover, in order to test the importance of DNA damage at telomeres in the ageing process, we investigated the presence of telomere-associated foci (TAF) in the gut and liver of mice, which have long telomeres and active telomerase but show increases of DNA damage foci frequencies in both tissues with age. We found an age-dependent increase in the frequencies of TAF in both the gut and liver. These data indicate that telomeres are important targets for genotoxic stress in vitro and in vivo with specific relevance for the induction of stress-induced senescence. TAF are persistent in stress-induced senescence We first tested whether persistent foci following X-ray irradiation were located at telomeres. We treated proliferation-competent human MRC5 fibroblasts and mouse embryonic fibroblasts (MEFs) with X-ray radiation (20 Gy and 10 Gy, respectively). As previously shown [7] , we confirmed that these levels of irradiation abolished cell proliferation and labelling indices for BrdU and Ki67, and caused increased activity of senescence-associated β-galactosidase (Sen-β-Gal) (results not shown). In order to test the sensitivity of telomeres to irradiation-induced DNA damage, we exposed MRC5 fibroblasts to increasing levels of X-ray irradiation ( Fig. 1a,b ). Frequencies of γH2A.X foci per nucleus increased with irradiation dose as expected ( Fig. 1a ). However, some DNA damage foci colocalized with telomeres as shown by immuno-FISH ( Fig. 1b,c and Supplementary Fig. S1 ). As the DNA damage foci we observe are the result of random DSB caused by irradiation, we have defined them as TAF, as opposed to telomere-induced foci, which are generally attributed to telomere uncapping. 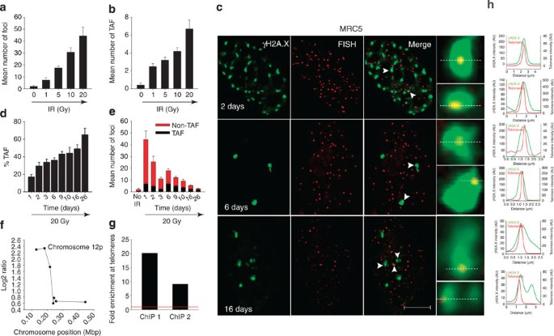Figure 1: TAF are persistent following X-ray-induced senescence in MRC5 fibroblasts with or without telomerase activity. (a) Total number of γH2A.X foci in human fibroblasts 1 day following irradiation with 1, 5, 10 and 20 Gy. Data are mean±s.e.m. ofn=15. (b) Total number of γH2A.X foci colocalizing with telomeres (TAF) in MRC5 fibroblasts 1 day after irradiation with 1, 5, 10 and 20 Gy. Data are mean±s.e.m. ofn=15. (c) Representative images of γH2A.X immuno-FISH in MRC5 fibroblasts 2, 6 and 16 days after 20 Gy. Images are Huygens (SVI) deconvolved Z projections of 3-μm stacks taken with a ×100 oil objective. White arrows indicate colocalization, and colocalizing foci are amplified in the right panel (amplified images are from single Z planes where colocalization was found). Scale bar=10 μm. (d) Percentage of γH2A.X foci colocalizing with telomeres (%TAF) in MRC5 fibroblasts up to 26 days after irradiation with 20 Gy. Data are mean±s.e.m. ofn=15. (e) Mean number of both TAF and non-TAF in MRC5 fibroblasts up to 26 days after irradiation with 20 Gy. Data are mean±s.e.m. ofn=15. (f) Enrichment of γH2AX at sub-telomeric regions was determined on chromosome 12p by ChIP followed by real-time PCR with previously independently validated primers at indicated distances from the chromosome end (10 days irradiated compared with non-irradiated MRC5 fibroblasts). Graph shows log2 ratios of irradiated and non-irradiated samples. Each PCR reaction was performed in triplicate. Data are mean from two independent ChIP experiments. (g) Enrichment of γH2AX at telomere repeats by real-time PCR. Graph represents fold enrichment of γH2AX at telomeric repeats between non-irradiated and 10 days irradiated cells for two independent ChIP experiments. Red line indicates non-irradiated control. (h) Graphs represent quantification of γH2A.X and telomere signals in selected regions of interest (dotted lines from 1c). Figure 1: TAF are persistent following X-ray-induced senescence in MRC5 fibroblasts with or without telomerase activity. ( a ) Total number of γH2A.X foci in human fibroblasts 1 day following irradiation with 1, 5, 10 and 20 Gy. Data are mean±s.e.m. of n =15. ( b ) Total number of γH2A.X foci colocalizing with telomeres (TAF) in MRC5 fibroblasts 1 day after irradiation with 1, 5, 10 and 20 Gy. Data are mean±s.e.m. of n =15. ( c ) Representative images of γH2A.X immuno-FISH in MRC5 fibroblasts 2, 6 and 16 days after 20 Gy. Images are Huygens (SVI) deconvolved Z projections of 3-μm stacks taken with a ×100 oil objective. White arrows indicate colocalization, and colocalizing foci are amplified in the right panel (amplified images are from single Z planes where colocalization was found). Scale bar=10 μm. ( d ) Percentage of γH2A.X foci colocalizing with telomeres (%TAF) in MRC5 fibroblasts up to 26 days after irradiation with 20 Gy. Data are mean±s.e.m. of n =15. ( e ) Mean number of both TAF and non-TAF in MRC5 fibroblasts up to 26 days after irradiation with 20 Gy. Data are mean±s.e.m. of n =15. ( f ) Enrichment of γH2AX at sub-telomeric regions was determined on chromosome 12p by ChIP followed by real-time PCR with previously independently validated primers at indicated distances from the chromosome end (10 days irradiated compared with non-irradiated MRC5 fibroblasts). Graph shows log2 ratios of irradiated and non-irradiated samples. Each PCR reaction was performed in triplicate. Data are mean from two independent ChIP experiments. ( g ) Enrichment of γH2AX at telomere repeats by real-time PCR. Graph represents fold enrichment of γH2AX at telomeric repeats between non-irradiated and 10 days irradiated cells for two independent ChIP experiments. Red line indicates non-irradiated control. ( h ) Graphs represent quantification of γH2A.X and telomere signals in selected regions of interest (dotted lines from 1c). Full size image As shown previously in MRC5 fibroblasts, only high doses of irradiation (20 Gy) can induce permanent cell arrest [7] , suggesting that TAF numbers might be the determining factor in cell-cycle arrest. While frequencies of non-TAF decreased rapidly following irradiation, the mean number of TAF per cell remained stable with time in human fibroblasts ( Fig. 1d,e ). These changes resulted in a time-dependent increase in the fraction of TAF ( Fig. 1d ). In young non-irradiated cells, as previously reported [18] , we found very low frequencies of cells positive for γH2A.X foci and overall low numbers of TAF ( Fig. 1e ). We also found that TAF were significantly larger than non-TAF at all time points analysed ( Supplementary Fig. S2 ), which is consistent with the reports that larger foci are persistent [19] . To assess independently the location of DDR proteins at telomeres following irradiation, we performed chromatin immunoprecipitation (ChIP) on cross-linked chromatin from MRC5 fibroblasts non-irradiated and 10 days after irradiation using an antibody against γH2A.X. We first confirmed the specificity of the ChIP by western blotting immunoprecipitated γH2A.X ( Supplementary Fig. S3 ) retrieved from phenol fraction following the ChIP assay. ChIP was followed by quantitative real-time PCR of sub-telomeric regions using a set of primers that had been previously validated for replicative senescent human fibroblasts and showed excellent concordance to ChIP–ChIP [20] . The results show robust enrichment of γH2A.X at sub-telomeric regions in chromosome 12 (10 days following irradiation when compared with non-irradiated controls) and that this enrichment increases abruptly in the direction of the end of the chromosome at 0.24 Mbp ( Fig. 1f ), similar to what was shown for replicative senescent fibroblasts. Moreover, in order to demonstrate that γH2A.X was in fact binding telomeric repeats and not just sub-telomeric regions, we performed quantitative real-time PCR for telomere repeats following γH2A.X ChIP. Our results show an average 14-fold enrichment of γH2A.X at telomere repeats 10 days after irradiation when compared with non-irradiated fibroblasts in two independent ChIP experiments ( Fig. 1g ). This confirms that colocalization observed by immuno-FISH is due to a physical association with telomeres and not mere proximity in the three-dimensional nuclear space. To determine that enrichment of γH2A.X foci at telomeres was not restricted to X-ray irradiation treatment, we have also incubated MRC5 fibroblasts with H 2 O 2 and neocarzinostatin (a protein–chromophore complex known for its anti-tumour activity). Similar to irradiation, we found evidence for both treatments of persistent DNA damage foci located at telomeres by immuno-FISH ( Fig. 2a,b ) at concentrations that induce cellular senescence ( Fig. 2c–f ). 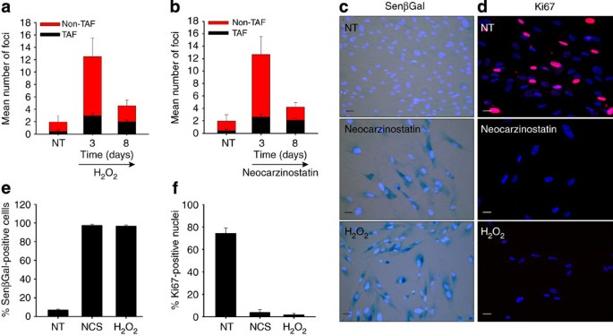Figure 2: TAF are persistent following H2O2- and neocarzinostatin-induced senescence in MRC5 fibroblasts. (a) Mean number of both TAF and non-TAF in MRC5 fibroblasts at 3 and 8 days after treatment for 1 h with hydrogen peroxide (400 μM in serum-free media). Data are mean±s.e.m.,n=15. (b) Mean number of both TAF and non-TAF in MRC5 fibroblasts at 3 and 8 days after treatment for 1 h with neocarzinostatin (80 ng ml−1). Mean±s.e.m.;n=15. (c) Representative images of Sen-β-Gal staining in non-treated (NT) MRC5 fibroblasts and 10 days after 1 h treatment with NCS (80 ng ml−1) and H2O2(400 μM) (light blue-DAPI; darker cytoplasmic blue- Sen-β-Gal). (d) Representative images of Ki67 staining in non-treated (NT) MRC5 fibroblasts and 10 days after 1 h treatment with NCS (80 ng ml−1) and H2O2(400 μM). (e) Quantification of mean number of Sen-β-Gal-positive cells and (f) Ki67-positive nuclei. Data are mean±s.e.m. (n=3). Scale bar: 20 μm. Figure 2: TAF are persistent following H 2 O 2 - and neocarzinostatin-induced senescence in MRC5 fibroblasts. ( a ) Mean number of both TAF and non-TAF in MRC5 fibroblasts at 3 and 8 days after treatment for 1 h with hydrogen peroxide (400 μM in serum-free media). Data are mean±s.e.m., n =15. ( b ) Mean number of both TAF and non-TAF in MRC5 fibroblasts at 3 and 8 days after treatment for 1 h with neocarzinostatin (80 ng ml −1 ). Mean±s.e.m. ; n =15. ( c ) Representative images of Sen-β-Gal staining in non-treated (NT) MRC5 fibroblasts and 10 days after 1 h treatment with NCS (80 ng ml −1 ) and H 2 O 2 (400 μM) (light blue-DAPI; darker cytoplasmic blue- Sen-β-Gal). ( d ) Representative images of Ki67 staining in non-treated (NT) MRC5 fibroblasts and 10 days after 1 h treatment with NCS (80 ng ml −1 ) and H 2 O 2 (400 μM). ( e ) Quantification of mean number of Sen-β-Gal-positive cells and ( f ) Ki67-positive nuclei. Data are mean±s.e.m. ( n =3). Scale bar: 20 μm. Full size image Overexpression of hTERT, the catalytic subunit of telomerase, has been shown to counteract telomere shortening, extend the replicative potential and prevent replicative senescence in cells [21] . To test the effects of hTERT overexpression on irradiation-induced telomere damage, we transfected proliferating-competent MRC5 human fibroblasts (PD25-30) with hTERT and subjected them to 20 Gy irradiation. MRC5 fibroblasts overexpressing hTERT showed high levels of telomerase activity, stable telomere length and extended replicative lifespan (results not shown and Ahmed et al . [22] ). We found that the presence of telomerase did not have a significant impact on numbers and percentage of TAF for up to 7 days after irradiation ( Fig. 3a–c ), cells still arrested irreversibly as shown by increased Sen-β-Gal activity and lack of the proliferation marker Ki67 ( Fig. 3d ). Accordingly, in MEFs that have long telomeres and telomerase activity, we found similar numbers and percentage of TAF as in human fibroblasts following irradiation ( Fig. 4a,b ). As in human fibroblasts, we observed that the frequencies of non-TAF decreased rapidly following irradiation and that the mean number of TAF per cell remained stable with time ( Fig. 4b,c ). 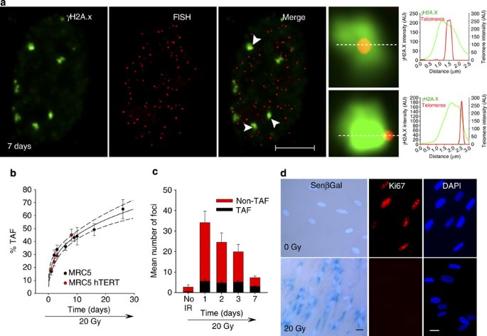Figure 3: Overexpression of hTERT in MRC5 fibroblasts does not suppress irradiation-induced cellular senescence and persistence of TAF. (a) Representative image of γH2A.X immuno-FISH in MRC5 fibroblasts overexpressing hTERT 7 days after 20 Gy. Images are Huygens (SVI) deconvolved Z projections of 3-μm stacks taken with a ×100 oil objective. White arrows indicate colocalization, and colocalizing foci are amplified in the right panel (amplified images are from single Z planes where colocalization was found). Graphs represent quantification of γH2A.X and telomere signals in selected regions of interest (dotted lines). Scale bar: 10 μm. (b) Comparison between % TAF in MRC5 fibroblasts with or without telomerase overexpression. Power curve (solid line) and 95% confidence intervals (dotted lines) are shown. Power curve best-fitted time-dependent increase in % TAF (R=0.9770,P=0.0001); Data are mean±s.e.m.;n=15. (c) Mean number of both TAF and non-TAF in MRC5 fibroblasts overexpressing hTERT up to 8 days after irradiation with 20 Gy; Mean±s.e.m.;n=15. (d) 20-Gy irradiation induces cellular senescence in MRC5 fibroblasts overexpressing hTERT. Representative images of staining for Sen-β-Gal (light blue: DAPI staining; cytoplasmic darker blue: Sen-β-Gal activity) and proliferation marker Ki67 (blue: DAPI, red: Ki67). Scale bar: 20 μm. Figure 3: Overexpression of hTERT in MRC5 fibroblasts does not suppress irradiation-induced cellular senescence and persistence of TAF. ( a ) Representative image of γH2A.X immuno-FISH in MRC5 fibroblasts overexpressing hTERT 7 days after 20 Gy. Images are Huygens (SVI) deconvolved Z projections of 3-μm stacks taken with a ×100 oil objective. White arrows indicate colocalization, and colocalizing foci are amplified in the right panel (amplified images are from single Z planes where colocalization was found). Graphs represent quantification of γH2A.X and telomere signals in selected regions of interest (dotted lines). Scale bar: 10 μm. ( b ) Comparison between % TAF in MRC5 fibroblasts with or without telomerase overexpression. Power curve (solid line) and 95% confidence intervals (dotted lines) are shown. Power curve best-fitted time-dependent increase in % TAF ( R =0.9770, P =0.0001); Data are mean±s.e.m. ; n =15. ( c ) Mean number of both TAF and non-TAF in MRC5 fibroblasts overexpressing hTERT up to 8 days after irradiation with 20 Gy; Mean±s.e.m. ; n =15. ( d ) 20-Gy irradiation induces cellular senescence in MRC5 fibroblasts overexpressing hTERT. Representative images of staining for Sen-β-Gal (light blue: DAPI staining; cytoplasmic darker blue: Sen-β-Gal activity) and proliferation marker Ki67 (blue: DAPI, red: Ki67). Scale bar: 20 μm. 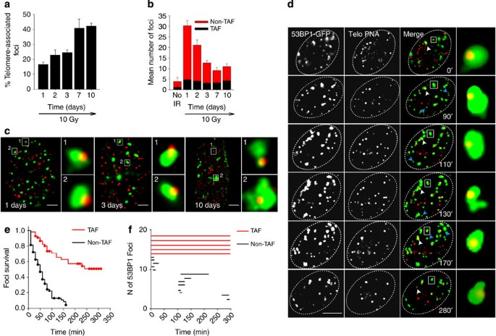Figure 4: Telomere-associated foci can be visualized in live MEFs and are longer lived than non-telomeric foci. (a) Percentage of 53BP1 foci colocalizing with telomeres (% TAF) in MEFs up to 10 days after irradiation with 10 Gy. (b) Mean number of both TAF and non-TAF in MEFs up to 10 days after irradiation with 20 Gy. (c) Representative images of Immuno-FISH using antibody against 53BP1 in fixed MEFs 1, 3 and 10 days after 10-Gy irradiation (red: telomeres, green: 53BP1). The white box indicates TAF and image on the right shows boxed image at higher magnification of a single Z plane. Images were taken with a Leica DM5500B fluorescence microscope. (d) Confocal time series of MEFs expressing AcGFP-53BP1c together with a PNA telomere probe 3 days after 10-Gy irradiation at the indicated times (min). Images are compressed stacks (maximum intensity projections) with a 4.5-μm focal depth. The white box indicates one TAF, which is permanent during the entire time series, and is shown at higher magnification on the right (single Z plane). White arrows indicate long-lived TAF and blue arrows short-lived non-TAF. (e) Kaplan–Mayer survival curves for AcGFP–53BP1c, which colocalize (TAF) or do not colocalize (non-TAF) with telomeres in MEFs 3 days after 10-Gy irradiation. The 200 foci were analysed from 8 cells. The Gehan–Breslow test shows a statistically significant difference between survival curves (P=<0.001). (f) Representative trace of AcGFP-53BP1c foci in one MEF for the indicated time 3 days after irradiation (10 Gy). Each bar represents the track of one individual focus recorded for the indicated time interval. 53BP1 foci colocalizing with telomere PNA probe are in red (TAF) and non-colocalizing foci are in black (non-TAF). A Zeiss LSM510 confocal microscope was used for live-cell imaging. Scale bars: 5 μm indand 10 μm inc. Full size image Figure 4: Telomere-associated foci can be visualized in live MEFs and are longer lived than non-telomeric foci. ( a ) Percentage of 53BP1 foci colocalizing with telomeres (% TAF) in MEFs up to 10 days after irradiation with 10 Gy. ( b ) Mean number of both TAF and non-TAF in MEFs up to 10 days after irradiation with 20 Gy. ( c ) Representative images of Immuno-FISH using antibody against 53BP1 in fixed MEFs 1, 3 and 10 days after 10-Gy irradiation (red: telomeres, green: 53BP1). The white box indicates TAF and image on the right shows boxed image at higher magnification of a single Z plane. Images were taken with a Leica DM5500B fluorescence microscope. ( d ) Confocal time series of MEFs expressing AcGFP-53BP1c together with a PNA telomere probe 3 days after 10-Gy irradiation at the indicated times (min). Images are compressed stacks (maximum intensity projections) with a 4.5-μm focal depth. The white box indicates one TAF, which is permanent during the entire time series, and is shown at higher magnification on the right (single Z plane). White arrows indicate long-lived TAF and blue arrows short-lived non-TAF. ( e ) Kaplan–Mayer survival curves for AcGFP–53BP1c, which colocalize (TAF) or do not colocalize (non-TAF) with telomeres in MEFs 3 days after 10-Gy irradiation. The 200 foci were analysed from 8 cells. The Gehan–Breslow test shows a statistically significant difference between survival curves ( P =<0.001). ( f ) Representative trace of AcGFP-53BP1c foci in one MEF for the indicated time 3 days after irradiation (10 Gy). Each bar represents the track of one individual focus recorded for the indicated time interval. 53BP1 foci colocalizing with telomere PNA probe are in red (TAF) and non-colocalizing foci are in black (non-TAF). A Zeiss LSM510 confocal microscope was used for live-cell imaging. Scale bars: 5 μm in d and 10 μm in c . Full size image TAF are longer-lived than non-TAF In order to establish whether telomeric location was necessary for foci persistence, we used kinetic live-cell microscopy. DNA damage foci lifespan was tracked by using a AcGFP-53BP1c fusion protein, which allowed us to quantitatively report DNA damage foci formation and degradation at the level of the individual focus [23] . We combined this with microbead-mediated incorporation of a fluorescently labelled PNA probe, which specifically tags telomere repeats. Owing to their stability, PNA probes can form PNA/DNA heteromultiplexes and allow visualization of telomeres in live cells for several hours [24] . To test whether the observed signals were indeed located at telomeres, after incorporation of a Cy3-labelled telomere probe in live cells, cells were fixed and hybridized with a FITC-labelled telomere probe. Results show that the majority of spots colocalize ( Supplementary Fig. S4a ). Metaphase spreads generated after microbead-mediated incorporation of a PNA telomere probe also reveal specific labelling of the ends of chromosomes ( Supplementary Fig. S4b ). For the first time, time-resolved live-cell microscopy allowed the kinetic tracking of telomeric and non-telomeric DNA damage foci independent from each other in the same cell after induction of senescence ( Fig. 4d ). We ensured proper tracking of individual foci by using a wide z-stack range (4.5 μm) and a high imaging frequency (every 10 min.). Videos were deconvolved using Huygens (SVI), and individual foci lifespan and colocalization with telomeres were tracked manually in MEFs starting at 3 days after irradiation. Live-cell microscopy detected similar numbers of telomeres in MEFs as FISH in fixed cells ( Supplementary Fig. S4a ). Moreover, no significant difference in average numbers of TAF per nucleus was observed by live-cell microscopy and by immuno-FISH at 3 days after 10 Gy irradiation (4.02±0.18 versus 3.1±0.28, P =0.07 two-tailed t -test). It is possible that incorporation of telomere PNA probes would induce TAF by eliciting dissociation of telomere-binding proteins from telomeres. However, we found in proliferating non-irradiated MEFs transfected with AcGFP-53BP1c fusion protein no evident induction of TAF after incorporation of PNA probes and generally very low number of 53BP1 DNA damage foci ( Supplementary Fig. S4b,c ). By manual tracking of foci, we constructed Kaplan–Maier survival curves for telomeric and non-telomeric foci in MEFs starting at 72 h after 10 Gy irradiation ( Fig. 4e ). The data show that all non-telomeric foci were short-lived, with a maximum lifespan of about 3 h. In contrast, only foci that colocalize with telomeric signals were able to survive for more than 3 h, and about 50% of TAF had a lifespan of >6 h ( Fig. 4e,f ). Previous work by our group had shown by live-cell imaging that foci lifespan increased in both replicative senescence and irradiation-induced senescence of human fibroblasts with half of all DDR foci being short-lived and dependent on oxidative stress [7] . Our recent data show that most, if not all, long-lived foci in stress-induced senescence colocalize with telomeres. This is in apparent contrast to a recent study [19] that reported no colocalization between TRF2 and 53BP1 10 days after irradiation in human fibroblasts. This inconsistency may be due to non-telomeric location of TRF2 as previously shown [25] . TAF increase with age irrespective of telomere length Our findings of persistent DNA damage foci at telomeres irrespective of telomerase activity led us to speculate whether random telomere damage could lead to accumulation of TAF in mouse tissues with age. So far, an age-dependent increase in the percentage of cells harbouring TAF has only been reported in skin fibroblasts from baboons [2] . An age-dependent increase in DNA damage foci in mice in several tissues, including enterocytes in intestinal crypts and hepatocytes (which we confirm here, Supplementary Fig. S5a,b ), together with increased oxidative stress markers has been reported [3] . Using high-resolution imaging of tissue sections, in depth Z stacking (a minimum of 40 optical slices with ×100 objective) followed by Huygens (SVI) deconvolution and manual quantification of colocalization by five independent analysts, we show that both liver hepatocytes and intestinal crypt enterocytes of C57BL/6 wild-type mice contain TAF and that the mean number of TAF per cell increases exponentially with age in both tissues ( Fig. 5a,c,d,f and g ). Moreover, the percentage of colocalizing foci per cell (%TAF) increases linearly with age in both tissues ( Fig. 5b,e ). Preliminary analysis of longitudinal gut sections revealed that most TAF-positive cells in the intestinal crypts of old animals were enterocytes in the transient amplifying zone of the crypts while enterocytes at the bottom of the crypts (where stem cells are located) generally have a low degree of colocalization (not shown). In both the intestine and liver, frequencies and localization of TAF-positive cells as demonstrated here ( Fig. 5 ) correspond well with frequencies of senescent cells in these tissues [3] , [26] . However, we found that the number of non-colocalizing foci per cell (non-TAF) does not increase significantly with age in either tissue ( Fig. 5i,j ), supporting the idea that TAF are persistent and accumulate with age, while non-TAF do not. 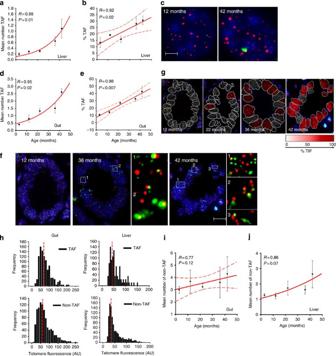Figure 5: Telomere-associated foci increase with age in the liver and small intestine of C57BL/6 mice. (a) Mean number of TAF per cell increases exponentially with age in hepatocytes from male C57BL/6 mice (exponential curve provided best fit withR=0.98;P=0.01) mean±s.e.m. ofn=3 per age group. (b) Percentage of TAF increase linearly with age in hepatocytes from male C57BJ6 mice (R=0.92;P=0.02) mean±s.e.m. ofn=3 per age group. (c) Representative immuno-FISH images of hepatocytes from 12-month- (left) and 42-month-old (right) mice. Green: γH2A.X; red: telomeres; blue: DAPI, Scale bar: 3 μm. (d) Mean number of TAF per cells increases exponentially with age in the small intestine enterocytes from male C57BL/6 mice (exponential curve provided best fit withR=0.95;P=0.02), mean±s.e.m. ofn=3 per age group. (e) Percentage of TAF increases linearly with age in enterocytes from male C57BL/6 mice (R=0.98;P=0.007) mean±s.e.m. ofn=3 per age group. (f) Representative immuno-FISH images in mice crypts at different ages. Boxed areas indicate colocalization between γH2A.X and telomeres, and are shown at higher magnification on the right (telomeres: red; γH2A.X: green and nucleus: DAPI; images are from one single Z plane), Scale bar: 20 μm. (g) Immuno-FISH images of 12-, 22-, 36- and 42-month-old mice colour coded according to degree of colocalization between γH2A.X and telomeres (white: low colocalization; red: high colocalization). (h) Histograms showing telomere intensity for telomeres colocalizing (bottom) or not colocalizing (top) with DNA damage foci in both the liver and gut from 36-month-old mice (n=3); red dotted line represents median intensity. Mann–Whitney test shows no significant difference in telomere intensities distribution between TAF and non-TAF for the small intestine (gut) (P=0.08) and a slight increase in liver telomere intensity in non-TAF (P=0.002). Intensity of 1,000 telomeres was analysed per condition. (i) Mean number of non-TAF per cell does not increase with age in small intestinal enterocytes from male C57BL/6 mice (linear curve provided best fit withR=0.77;P=0.12) mean±s.e.m. ofn=3 per age group. (j) Mean number of non-TAF per cell does not increase with age in hepatocytes from male C57BL/6 mice (exponential curve provided best fit withR=0.86;P=0.07) mean±s.e.m. ofn=3 per age group. Figure 5: Telomere-associated foci increase with age in the liver and small intestine of C57BL/6 mice. ( a ) Mean number of TAF per cell increases exponentially with age in hepatocytes from male C57BL/6 mice (exponential curve provided best fit with R =0.98; P =0.01) mean±s.e.m. of n =3 per age group. ( b ) Percentage of TAF increase linearly with age in hepatocytes from male C57BJ6 mice ( R =0.92; P =0.02) mean±s.e.m. of n =3 per age group. ( c ) Representative immuno-FISH images of hepatocytes from 12-month- (left) and 42-month-old (right) mice. Green: γH2A.X; red: telomeres; blue: DAPI, Scale bar: 3 μm. ( d ) Mean number of TAF per cells increases exponentially with age in the small intestine enterocytes from male C57BL/6 mice (exponential curve provided best fit with R =0.95; P =0.02), mean±s.e.m. of n =3 per age group. ( e ) Percentage of TAF increases linearly with age in enterocytes from male C57BL/6 mice ( R =0.98; P =0.007) mean±s.e.m. of n =3 per age group. ( f ) Representative immuno-FISH images in mice crypts at different ages. Boxed areas indicate colocalization between γH2A.X and telomeres, and are shown at higher magnification on the right (telomeres: red; γH2A.X: green and nucleus: DAPI; images are from one single Z plane), Scale bar: 20 μm. ( g ) Immuno-FISH images of 12-, 22-, 36- and 42-month-old mice colour coded according to degree of colocalization between γH2A.X and telomeres (white: low colocalization; red: high colocalization). ( h ) Histograms showing telomere intensity for telomeres colocalizing (bottom) or not colocalizing (top) with DNA damage foci in both the liver and gut from 36-month-old mice ( n =3); red dotted line represents median intensity. Mann–Whitney test shows no significant difference in telomere intensities distribution between TAF and non-TAF for the small intestine (gut) ( P =0.08) and a slight increase in liver telomere intensity in non-TAF ( P =0.002). Intensity of 1,000 telomeres was analysed per condition. ( i ) Mean number of non-TAF per cell does not increase with age in small intestinal enterocytes from male C57BL/6 mice (linear curve provided best fit with R =0.77; P =0.12) mean±s.e.m. of n =3 per age group. ( j ) Mean number of non-TAF per cell does not increase with age in hepatocytes from male C57BL/6 mice (exponential curve provided best fit with R =0.86; P =0.07) mean±s.e.m. of n =3 per age group. Full size image It is not clear at present whether TAF as seen in tissues of ageing mice are the result of telomere shortening or random telomeric damage. Mouse gut is a highly proliferative tissue, and an age-dependent decrease in telomere length in C57BL/6 mice intestine has been reported [3] , [27] , which can increase the probability of telomere uncapping and detection by DDR proteins. To test whether the presence of TAF could be explained by telomere shortening, we quantified telomere intensity of both colocalizing (TAF) and non-colocalizing (non-TAF) telomeres. In old mice intestinal crypts, we found no statistically significant difference between telomere length distributions in TAF and non-TAF (Mann–Whitney test, P =0.08) and a slight increase in median telomere length in the liver TAF (Mann–Whitney test, P =0.002) ( Fig. 5h ), suggesting that telomere length is not the sole defining factor in the induction of TAF. Our results show for the first time that TAF increases with age in mouse liver. As very low frequencies of proliferating hepatocytes were observed at any age, we hypothesize that oxidative stress may be responsible for increased telomere damage. In effect, we have previously reported that hepatocytes containing DDR foci were also positive for oxidative stress markers [26] . Maintenance of genomic stability requires that ends of chromosomes possess special characteristics, which make them distinct from DSBs. While these characteristics are essential for prevention of telomere end-to-end fusions, our results suggest that they might have detrimental consequences in terms of DNA repair capacity following random DNA damage whether it is caused endogenously by oxidative stress or exogenously by DNA-damaging agents. Previous work has attributed a key role for TRF2 in the distinction between telomeres and DSBs. Displacement of TRF2 from telomeres by overexpression of TRF2 ΔBΔM or conditional deletion of TRF2 in mouse cells has been shown to result in ligase-IV-dependent telomere fusions [16] , [28] , [29] . It has also been described in vitro that TRF2 and its binding partner RAP1 are required to prevent NHEJ-dependent telomeric DNA fusions by inhibiting DNA-PK and ligase-IV-mediated end joining [17] . Telomere-binding proteins may also impact on regions adjacent to telomere repeats. This DSB repair inhibition was demonstrated in Saccharomyces cerevisiae where signalling from DNA breaks was inhibited up to 0.6 kb from telomeres [30] . Thus, while our Immuno-FISH results point to DDR occurring specifically at telomeric repeats following genotoxic stress, it is possible that regions adjacent to telomeres may have been affected. However, it is methodologically difficult to establish the exact position of the DNA DSB as it has been shown that telomere-induced foci extend well beyond telomere repeats. In fact, ChIP–Chip assays on replicatively senescent cells detected spreading of γH2A.X hundreds of kilobases in several chromosome ends [9] , [20] similar to our results in chromosome 12p following irradiation. While our data show direct binding of γH2A.X to telomeric repeats, we are unable to determine experimentally whether a persistent DNA damage is occurring at the chromosome end or within telomeric repeats. For that reason, several scenarios can be proposed to explain our data: it is possible that genotoxic stress contributes to the loss of telomere loop (t-loop) conformation and leads to a DDR at telomere ends. T-loop has been hypothesized to be maintained by binding of shelterin components [10] , [31] and dependent on telomere length [32] . Our data point to a persistent DDR occurring irrespectively of telomere length following genotoxic stress and during ageing in mice, which would be inconsistent with the idea of short telomeres inducing loss of protective cap. However, it is still possible that random oxidative damage to telomere repeats will affect binding ability to shelterin components as supported by in vitro assays, which show that binding of TRF1 and TRF2 to telomeres is reduced by oxidative DNA damage [33] . An additional scenario has been proposed by Cesare et al . [14] They demonstrated in cancer cells that a spontaneous DDR at telomeres could occur in the absence of chromosome fusions, suggesting the existence of an intermediary state of telomere capping, which retains sufficient TRF2 or other shelterin components to suppress NHEJ without inhibiting a DDR at telomere ends [14] . This scenario, the authors have shown, can occur partly independent of telomere length in ALT (alternative lengthening of telomeres)-positive cancer cell lines [14] . This could explain persistent DDR at telomeres irrespectively of length in the absence of NHEJ. A final scenario is that random DNA damage generated by genotoxic stress occurs within telomeric repeats and does not lead to recognition of chromosome terminal ends by DDR. Shelterin components (such as TRF2) would then act to repress NHEJ in telomeric repeats throughout their length, while allowing a persistent DDR. This would be consistent with in vitro data showing that telomeric repeats are resistant to NHEJ [17] and that a DDR can occur in long telomeres concomitantly with inhibition of NHEJ [14] . Persistence of TAF following X-ray irradiation-induced senescence were observed independently by d'Adda di Fagagna's group and the authors suggest that TRF2 plays a role in inhibition of NHEJ repair (ref. 34 ) Our data also suggest that telomeric regions, despite occupying a minute fraction of the genome, are favoured targets for random DNA damage. In fact, previous work has demonstrated that telomeres are particularly sensitive to oxidative stress when compared with the bulk of the genome [15] and less efficiently repaired when subjected to single-stranded breaks and UV-induced damage [35] . It has been argued that this sensitivity to single-stranded breaks might be due to the fact that telomeric repeats contain guanine triplets that are remarkably sensitive to oxidative modifications [36] , [37] . These factors, coupled with the reported protection of telomeres from repair activities, may contribute to their specific targeting and persistent damage as a consequence of genotoxic stress. However, further work needs to be conducted in order to elucidate the characteristics of telomeres that make them particularly susceptible to damage. We conclude that persistent telomere-associated damage is a frequent outcome of genotoxic stress and a component of stress-induced senescence, which is independent of telomerase activity and telomere length, and may contribute to age-related decline in the tissue function. This highlights the relevance of telomeres as targets of stress-related ageing. Cell culture and treatments Human embryonic lung MRC5 fibroblasts were obtained from ECACC (Salisbury, UK) and grown in DMEM (Sigma, Dorset, UK) supplemented with 10% heat-inactivated foetal calf serum, penicillin/streptomycin and 2 mM glutamine under atmospheric oxygen conditions (air plus 5% CO 2 ). Mouse embryonic fibroblasts (MEFs) were obtained from C57BL/6 wild-type mice and cultured in DMEM (Sigma) plus 10% FSC, penicillin/streptomycin and 2 mM glutamine at 3% ambient oxygen in a 3-gas cell culture incubator (Zapf Instruments, Sarstedt, Germany). MRC5 fibroblasts (PD 25–30) were transfected retrovirally with the catalytic subunit of telomerase hTERT as described [22] . MEFs at 50% confluency were transiently transfected with a 53BP1 reporter protein using plasmid pG-AcGFP-53BP1c using Fugene6 (Roche, Welwyn, UK) at a ratio of 3 μl fugene: 2 μg DNA following the manufacturer's instructions. Stress-induced senescence in MRC5 fibroblasts was induced by X-ray irradiation with 20 Gy, neocarzinostatin (80 ng ml −1 ) for 1 h or H 2 O 2 (400 μM) in serum-free media for 1 h. Following treatment, culture medium was refreshed. Senescence was induced in MEFs by X-ray irradiation with 10 Gy. Animals Three male C57BL/6 mice per age group (3, 12, 22, 36 and 42 months) were killed. Tissues were immediately perfusion fixed. Formalin-fixed paraffin-embedded 3-μm sections were prepared from the liver and gut. All work was complied with the guiding principles for the care and use of laboratory animals. The project was approved by the Faculty of Medical Sciences Ethical Review Committee, Newcastle University. Project licence number 60/3864. Immunofluorescence For immunostaining, cells grown on sterile coverslips were fixed in 2% paraformaldehyde and incubated with a primary antibody for 1 h at room temperature, followed by either an Alexa Fluor® 594 or Alexa Fluor® 488 secondary antibody (Invitrogen) 45-min incubation. Antibodies used: rabbit polyclonal anti-Ki67 antibody (ab15580; 4 μg ml −1 Abcam), mouse monoclonal anti-γ-H2A.X antibody (AB10022; 0.25 μg ml –1 Upstate Millipore), rabbit monoclonal anti-γ-H2A.X IgG (S139) (#9718; 0.4 μg ml –1 Cell Signaling), rabbit polyclonal anti-53BP1 antibody (#4937; 0.2 μg ml –1 Cell Signaling) and rabbit polyclonal anti-53BP1 (NB100-904 4 μg ml –1 Novus Biologicals). Immuno-FISH Immuno-FISH was performed as described [18] . Briefly, cells grown on sterile coverslips were fixed with 2% paraformaldehyde and incubated with anti- γ-H2A.X (Upstate Biotechnology) or anti-53BP1 (Cell Signaling) antibodies for 1 h at room temperature as described above. After application of the secondary antibody, cells were washed with PBS and FISH was performed. 20 μl of Cy-3-labelled telomere specific (C3TA2)3 peptide nucleic acid (PNA) probe (4 ng μl −1 ) (Panagene) was applied to the cells followed by co-denaturation at 80 °C and hybridization for 2 h at room temperature in the dark. Cells were then washed three times for 10 min with wash buffer made from 70 ml formamide (70%), 30 ml SSC 2% (3 ml stock SSC 20%+27 ml H 2 0) and three times for 5 min with TBS-Tween 0.05%. Cells were incubated with 4,6-diamidino-2-phenylindole (DAPI), mounted and imaged using a Leica DM5500B fluorescence microscope. In depth Z stacking was used (images were captured as stacks separated by 0.247 μm with ×100 objective) followed by Huygens (SVI) deconvolution. For Immuno-FISH in formalin-fixed paraffin-embedded liver and gut mice tissues, sections were hydrated by incubation in 100% Histoclear, 100, 95 and 70% methanol for 5 min (twice) and finally in distilled water for 5 min (twice). For antigen retrieval, the slides were placed in 0.1 M citrate buffer and heated until boiling for 10 min. After cooling down to room temperature, the slides were washed twice with distilled water for 5 min. After blocking in normal goat serum (1:60) in BSA/PBS, primary antibody (rabbit γ-H2A.X 1:250) was applied and incubated at 4 °C overnight. The next day, slides were washed three times in PBS, incubated with secondary antibody for 30 min, washed three times in PBS and incubated with Avidin DCS (1:500) for 20 min. Following incubation, slides were washed three times in PBS and dehydrated with 70, 90 and 100% ethanol for 3 min each. Sections were denatured for 5 min at 80 °C in hybridization buffer (70% formamide (Sigma), 25 mM MgCl 2 , 1 M Tris pH 7.2, 5% blocking reagent (Roche)) containing 2.5 μg ml −1 Cy-3-labelled telomere specific (CCCTAA) peptide nuclei acid probe (Panagene), followed by hybridization for 2 h at room temperature in the dark. The slides were washed twice, for 15 min each, with 70% formamide in 2×SSC, followed by 2×SSC and PBS washes for 10 min. Sections were incubated with DAPI, mounted and imaged. In depth Z stacking was used (a minimum of 40 optical slices with ×100 objective) followed by Huygens (SVI) deconvolution. Crosslinked ChIP assay Crosslinked ChIP assay was carried out using 100-μg crosslinked chromatin prepared from control or irradiated MRC5 fibroblasts (10 days after 20 Gy) as described previously [38] . Antibody used for immunoprecipitation raised against γH2A.X was purchased from Upstate Biotechnology. Isotype and species-matched control ChIP grade IgG was obtained from Abcam. The 10 μg of each antibody were used in each ChIP reaction. Real-time PCR Primers used for the detection of relevant sub-telomeric sequences of chromosome 12p were as published in ref. 20 . Real-time PCR specific for telomeric repeats was performed as described in ref. 39 . Briefly, 4 μl of ChIP eluate was added to a final volume of 13 μl quantitative PCR reaction containing 6.5 μl Jumpstart SYBR master mix (Sigma) and 10 pmol appropriate primer mix. Telomere and sub-telomere PCR reaction conditions were: 10 s at 95 °C followed by 40 cycles of 10 s at 95 °C, 30 s at 55 °C and 30 s at 72 °C followed by ABI7500 Fast Real-Time PCR System machine predetermined melt curve analysis (Applied Biosystems). Each PCR reaction was performed in triplicate from two independent ChIP experiments. All reactions were normalized to the control antibody and fold enrichment above background was calculated using the following equation: (1/(2A)) ×100. The values were then adjusted to the values of total input and expressed as log to the base 2. Extraction of immunoprecipitated γH2A.X from phenol fraction Following reversal of crosslinks after the ChIP assay, eluate was mixed with equal amount of phenol and centrifuged at 13,000 r.p.m. for 5 min. DNA-containing fraction was removed, cleaned up and used in PCR, whereas 500 μl of phenol was mixed with concentrated HCl (final concentration of 0.4 M) and ten volumes of acetone. This mix was allowed to precipitate at −80 °C overnight. Precipitated histones were pelleted at 3,500 r.p.m. for 20 min at 4 °C. The pellets were washed three times in acetone, vacuum dried and resuspended in 10 μl of 8 M urea/10% β-mercaptoethanol. Samples were heated to 65 °C for 10 min, then 10 μl of SDS–polyacrylamide gel electrophoresis loading buffer was added, mixed and heated to 100 °C for 5 min before loading on a 12% SDS–polyacrylamide gel electrophoresis gel. Western blots were carried out using routine protocol from this point onwards. Telomere PNA probes incorporation and live-cell imaging Incorporation of telomere-specific PNA probe by glass beads was performed as described [24] . Briefly, the Cy-3-labelled telomere-specific (C3TA2)3 peptide nucleic acid (PNA) probe (Panagene) was dissolved in 80 mM KCl, 10 mM K 2 PO 4 , 4 mM NaCl, pH 7.2, to a final concentration of 1 μM. MEFs were grown in glass-bottomed dishes and PNA probe was pipetted onto the culture. A 0.12 g of 75 μm alkali-washed glass beads (Sigma) were carefully and evenly sprinkled onto the surface of the dish, and cells were allowed to recover for 2 h in DMEM (10% FSC). To confirm that PNA probe was located at telomeres, following Cy-3-labelled telomere-specific PNA probe incorporation in live MEFs, cells were fixed in 2% paraformaldehyde and FISH was performed, as described above, using a FITC-labelled telomere specific (C3TA2)3 peptide nucleic acid (PNA) probe (Panagene). For live-cell timelapse microscopy of the 53BP1 reporter and PNA probe, a Zeiss LSM510 confocal microscope equipped with a Solent incubator (Solent Scientific) at 37 °C with humidified 5% CO 2 , using a ×63 (NA=1.4) objective, was used as described [23] . MEFs were plated in Iwaki glass-bottomed dishes (Iwaki) and imaged using a 63×1.3 NA oil objective. AcGFP-53BP1c foci and telomere PNA probes were tracked manually using ImageJ ( http://rsb.info.nih.gov/ij/ ). Metaphase spreads Metaphase spreads from MEFs were prepared by treatment of subconfluent cells with 10 μg ml −1 colcemid for 2 h at 37 °C, followed by 60 mM KCl for 15 min at room temperature and fixation in ethanol:acetic acid (3:1) as described in ref. 18 . Slides were air-dried, stained with DAPI and imaged using a Leica DM5500B fluorescence microscope. Senescence-associated β-galactosidase staining For senescence-associated β-galactosidase staining, cells were fixed with 2% formaldehyde in PBS for 5 min and stained as described in ref. 40 . Briefly, following fixation, cells were washed once with PBS and incubated at 37 °C for 16 h in freshly prepared senescence-associated β-galactosidase staining solution containing 2 mM magnesium chloride, 150 mM sodium chloride, 40 mM citric acid, 12 mM sodium phosphate dibasic, 5 mM potassium ferrocyanide, 5 mM potassium ferricyanide and 1 mg l −1 5-bromo-4-chloro-3-inolyl-β-d-galactoside (X-Gal) at pH 6.0. Following staining, nuclei were stained with DAPI and cells were imaged. Statistical analyses We conducted two-tailed t -tests, linear and non-linear regression analysis, and Gehan–Breslow test using Sigma Plot vs11.0. Wilcoxon–Mann–Whitney tests were conducted using IBM SPSS Statistics 19. How to cite this article: Hewitt, G. et al . Telomeres are favoured targets of a persistent DNA damage response in ageing and stress-induced senescence. Nat. Commun. 3:708 doi: 10.1038/ncomms1708 (2012).